Bond competition and phase evolution on the IrTe2surface Compounds with incommensurate structural modulations have been extensively studied in last several decades. However, the relationship between structurally incommensurate/commensurate phases and associated electronic states remains enigmatic. Here we report the coexisting of complex incommensurate structures and highly unusual electronic roughness on the surface of in situ cleaved IrTe 2 by using scanning tunnelling microscopy/spectroscopy, corroborated with extensive density-functional theory calculations. This behaviour is traced to structural instability, which induces a structural transition from a trigonal to a triclinic lattice below transition temperature, giving rise to the formation of unidirectional structural modulations with distinct wavelengths, accompanied by the opening of a ‘pseudo’-gap in the surface layer. With further cooling the surface adopts a structure that reflects an ~6 × periodicity that is different from the bulk 5 × periodicity. Calculations show that the structure distortion is not associated with a charge density wave, but is rather associated with Te p-electron bonding. Competition between ground states often leads to the realization of new states with properties that cannot be readily anticipated from those of the original states. One example is the Frenkel–Kontorova model (chain of atoms on a simple periodic substrate), where a competition between two periodicities leads to an exceedingly complex structural evolution, including solitons, and a devils staircase [1] . In this case a simple uniform Hamiltonian leads to ground states that are highly inhomogeneous on all length scales. Structural competition and modulations are also of importance in technological materials ranging from superconductors near density waves to piezoelectric morphotropic phase boundary systems. In bulk systems, coupling of a frustrated structural instability of a metal to the electronic structure can lead to remarkably subtle ground states, as exemplified by the Verwey metal-insulator transition of Fe 3 O 4 where solution of the low-temperature structure has attracted long-standing interest but was only recently elucidated [2] . The case of frustration between bulk and surface structural transitions in materials with interesting electronic coupling is less studied, but may be more amenable to detailed investigation since the exposed surface allows direct probing of the interplay of spatial inhomogeneity and electronic structure particularly using scanning probes. In fact, spatially resolved studies are particularly useful for such systems due to the central role of inhomogeneity in these emergent states. We focus on the 5d transition metal ditelluride IrTe 2 using a combination of scanning tunnelling microscopy, which provides local structural information, and spectroscopy, which provides local electronic information. We show that this system does exhibit a complex surface structure on extended length scales, incommensurate with the bulk structure, and that this leads to a spatially inhomogeneous electronic reconstruction. IrTe 2 at above T s ~270 K is a metal with a high-symmetry layered trigonal structure. As it is cooled through T s it undergoes a metal–metal transition to a complex reconstructed 5 × 1 × 5 structure [3] . This material, when stabilized by alloying or intercalation, is superconducting [4] , [5] , suggesting substantial electron–phonon coupling. In the high-temperature trigonal phase (HT), the Ir ions form an equilateral-triangular lattice in the ab plane with edge-sharing IrTe 6 octahedra forming layers stacked along the c axis (see Supplementary Fig. 1a ). The low-temperature triclinic phase (LT) of IrTe 2 has strong aspect of a unidirectional modulated superstructure and also involves rebonding of Te atoms between layers. While the phase transition was initially discussed as a density wave [5] , more recent studies, including our first-principles calculations discussed below, show that it is not a charge density wave (CDW) but is instead a consequence of competition between Te–Ir, covalent/ionic and Te–Te covalent p-electron bonding [6] , [7] , [8] , [9] . Both the HT and LT phases of IrTe 2 show significant three-dimensional electronic structures reflecting interactions (and in the case of the LT phase, bonding) between adjacent CdI 2 structure layers, which is very different from most layered dichalcogenides, which are generally more two dimensional and show real CDW instabilities [10] . Several scanning tunnelling microscope (STM) studies [11] , [12] have been reported recently on IrTe 2 , but the relationship between the structural and electronic properties remains to be fully elucidated. In any case, the fact that the transition is associated with Te–Te bonding with interlayer bonds suggests that the surface may favour a different pattern than the bulk leading to a competition. Moreover, a change of the modulation from 1/5 to 1/6 is observed by Se doping [9] or the further cooling [12] , both suggesting that the intrinsic ground state of IrTe 2 is a 1/6 modulation. Here we report observation of coexisting complex incommensurate structures, presumably due to bond competition, based on atomic-resolved imaging of nanophase domains. The structural transition, which is mainly a distortion of the Te sublattice in this compound, produces multiple structural modulations on surface, inducing a strong reconstruction of Te p bands. We find this to be associated with enhanced electronic roughness in these coexisting structures. Although the bulk transition is strongly first order, we find that the electronic roughness at the surface is significantly temperature dependent and vanishes in the LT phase when the temperature is close to the critical temperature. Specifically, the surface electronic structure is characterized by a position-dependent partial gapping. As the critical temperature is approached with cooling, this electronic roughness vanishes and the partial gap further develops into a more complete gap. Accompanied with the full gap formation at 4.2 K, the incommensurate modulation at 77 K changes to a homogeneous commensurate 1/6 modulation, suggesting that the intrinsic ground state of IrTe 2 is a 1/6 modulation. We also report density-functional theory (DFT) calculations, showing that the structural modulations are not induced by Fermi surface nesting, suggesting that the interplay between structure instability and electronic structure reconstruction does lead to electronic inhomogeneity in this system consistent with the observations. STM study of an incommensurate LT phase of IrTe 2 surface Unidirectional superlattice/modulations are clearly seen in our STM topographic images taken at 77 K ( Fig. 1a ). The images show the multiple unidirectional modulations with distinct wavelengths. In addition to the unidirectional modulations, some one-dimensional deep trenches, run parallel to each other across the surface as seen in the zoomed-in atomically resolved image ( Fig. 1b ). We performed two-dimensional Fourier analysis of the atomically resolved STM images to characterize these patterns. The Fourier transform of Fig. 1b (in Fig. 1c ) reveals a series of fractional spots along the b′ direction in reciprocal space, implying the existence of multiple modulations instead of the regular hexagonal lattice (atomic lattice marked by blue circles) or a modulated structure derived directly from the bulk. To better visualize the fractional spots, we enlarge the central reciprocal area and show modulation spots in the bottom panel. The measured periodicities λ 1Q of modulations, are about 2.75 a 0 , 4.22 a 0 , 7.58 a 0 and 9.26 a 0 , corresponding to q 1Q ~0.364 Q 0 , 0.237 Q 0 , 0.132 Q 0 and 0.108 Q 0, respectively, where Q 0 is the Bragg vector. Here, a 0 represents the Te–Te atomic distance along the nonmodulated direction ( b axis), which is equal to 3.82 Å at 77 K. (see Supplementary Fig. 2 ). We label these incommensurate modulations, respectively, as q 1 , q 2 , q 3 and q 4 for simplicity. We enlarge three areas (marked as red rectangles in Fig. 1b ) and exhibit high-resolution (HR) images in three panels in Fig. 1d for superlattices of q 1 , q 3 and q 4 . The unit cells (UCs)of these incommensurate modulations are highlighted by blue parallelograms in each panel. Take 7.58 a 0 modulation for example, although the periodicity is 7.58 a 0 , each UC involves eight atomic rows, giving rise to an ‘8 times’-like modulation in the STM images [12] . As a consequence, the mean distance between rows at 77 K is about 0.95 a 0 , smaller than that value along the direction of the b axis (see Supplementary Fig. 2 and Note 1 for details ). By using one-dimensional fast fourier transform phase analysis, coexisting incommensurate domain structures are illustrated based on the phase profile plot in Supplementary Figs 3 and 4 (see Supplementary Note 2 for details ). 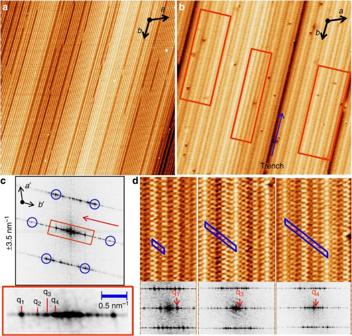Figure 1: High-resolution STM images for surface modulations at 77 K. (a) A typical topographic image of IrTe2surface taken at 77 K, where a unidirectional superlattice appears on this surface. The setup conditions for imaging were a sample-bias voltage of 200 mV, a tunnelling current of 20 pA with the scan range of 240 × 240 nm2. (b) Atomically resolved image of IrTe2surface at 77 K, instead of showing a basically hexagonal lattice of surface atoms, displays clear signs of the formation of surface unidirectional modulations. The scan range is 36 × 36 nm2with a bias of −200 mV and a tunnelling current of 0.05 nA. (c) Fourier transform image (upper) of theband a zoom-in enlargement showing the details of fractional spots (bottom), which displays surface modulations with multiple periodicities of 2.75 × (q1), 4.22 × (q2), 7.58 × (q3) and 9.26 × a0(q4). (d) A series of zoom-in STM images showing the modulations with different periodicities of 2.75 × , 7.58 × and 9.26 × (from left to right), respectively. The surface unit cells are marked by a blue parallelogram, depending on its orientation. The sizes of images: 3.6 × 6.4 nm2, 5.1 × 6.4 nm2and 5.1 × 6.4 nm2from left to right, respectively. Figure 1: High-resolution STM images for surface modulations at 77 K. ( a ) A typical topographic image of IrTe 2 surface taken at 77 K, where a unidirectional superlattice appears on this surface. The setup conditions for imaging were a sample-bias voltage of 200 mV, a tunnelling current of 20 pA with the scan range of 240 × 240 nm 2 . ( b ) Atomically resolved image of IrTe 2 surface at 77 K, instead of showing a basically hexagonal lattice of surface atoms, displays clear signs of the formation of surface unidirectional modulations. The scan range is 36 × 36 nm 2 with a bias of −200 mV and a tunnelling current of 0.05 nA. ( c ) Fourier transform image (upper) of the b and a zoom-in enlargement showing the details of fractional spots (bottom), which displays surface modulations with multiple periodicities of 2.75 × (q 1 ), 4.22 × (q 2 ), 7.58 × (q 3 ) and 9.26 × a 0 (q 4 ). ( d ) A series of zoom-in STM images showing the modulations with different periodicities of 2.75 × , 7.58 × and 9.26 × (from left to right), respectively. The surface unit cells are marked by a blue parallelogram, depending on its orientation. The sizes of images: 3.6 × 6.4 nm 2 , 5.1 × 6.4 nm 2 and 5.1 × 6.4 nm 2 from left to right, respectively. Full size image To get an insight into the electronic structure associated with these incommensurate domains, we further study the energy dependence of these modulated structures. The standard variation roughness analysis was performed with a set of different sample biases, shown in Supplementary Figs 5 and 6 . The analysis has clearly demonstrated that there is a strong energy dependence of the surface roughness, which implies that an electronic inhomogeneity may be associated with these incommensurate modulated structures (see Supplementary Note 3 for details ). Focusing on a region with q 3 modulation, Fig. 2a shows an atomic-resolved STM image at −0.2 V. A repeated surface UC is defined along the a axis. To illustrate the inner structure of the UC, we zoom into a small area with the size of 4 × 4 nm. Imaging at both positive and negative sample biases will help to elucidate the spatial electronic contribution from structural topography. By placing two constant-current images taken at +0.2 V ( Fig. 2b ) and −0.2 V ( Fig. 2c ), we are able to obtain insight into the atomic structure and electronic modulation in a single surface UC. For a better picture of the electronic spatial variation, a spectroscopic survey was taken, consisting of 25 differential tunnelling conductance spectra (d I/ d V versus V ) measurements. 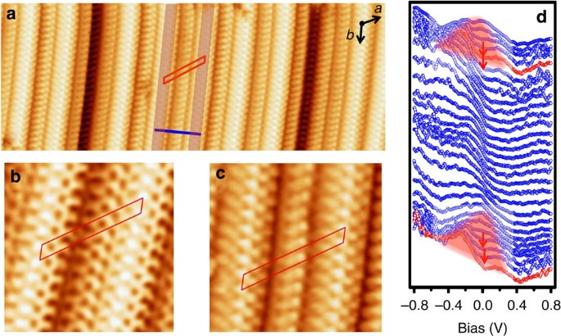Figure 2: Electronic roughness and the opening of a ‘pseudo’-gap within a 7.58 a0superlattice unit cell. (a) Atomically resolved image of IrTe2surface at 77 K, displays clear signs of surface modulation periodicity of 7.58 a0. The surface unit cells are marked by a red parallelogram. The setup conditions for imaging were a sample-bias voltage of −200 mV, a tunnelling current of 0.1 nA with the scan range of 24 × 9 nm2. (b,c) Zoom-in highly resolved STM images at +200 mV (b) and −200 mV (c) sample biases, reveal the atomic structure within a UC of surface superlattice. (d) A series of dI/dVspectra acquired along the blue line ina. The highlighted red curves locate on the top of brightest atomic rows, exhibiting electronic states suppression around the Fermi level. The red shaded area highlights the evolution from a ‘bump’ in local density of states (LDOS) to a suppressed zero-bias DOS. Here, all spectra were taken at 77 K with a bias of −100 mV and a tunneling current of 0.1 nA. Bias-modulation amplitude was set to 5 mVr.m.s.. Figure 2: Electronic roughness and the opening of a ‘pseudo’-gap within a 7.58 a 0 superlattice unit cell. ( a ) Atomically resolved image of IrTe 2 surface at 77 K, displays clear signs of surface modulation periodicity of 7.58 a 0 . The surface unit cells are marked by a red parallelogram. The setup conditions for imaging were a sample-bias voltage of −200 mV, a tunnelling current of 0.1 nA with the scan range of 24 × 9 nm 2 . ( b , c ) Zoom-in highly resolved STM images at +200 mV ( b ) and −200 mV ( c ) sample biases, reveal the atomic structure within a UC of surface superlattice. ( d ) A series of d I/ d V spectra acquired along the blue line in a . The highlighted red curves locate on the top of brightest atomic rows, exhibiting electronic states suppression around the Fermi level. The red shaded area highlights the evolution from a ‘bump’ in local density of states (LDOS) to a suppressed zero-bias DOS. Here, all spectra were taken at 77 K with a bias of −100 mV and a tunneling current of 0.1 nA. Bias-modulation amplitude was set to 5 mV r.m.s. . Full size image Figure 2d shows the d I/ d V spectra acquired within one UC (marked by a blue line in Fig. 2a ), all exhibit similar asymmetric line shapes. However, suppression around the Fermi level ( E F ) gradually develops into a ‘pseudo’-gap feature (shading by red colour in Fig. 2d ), while the rest of the d I/ d V curves exhibit a ‘bump’ at E F in density of states (DOS). Such gap-like features only open periodically at the location corresponding to ‘bright’ atomic rows, shaded by pink stripes in Fig. 2a . The suppression around E F in DOS of IrTe 2 was also observed in PES measurements by Ootsuki et al. [8] , explained by band narrowing due to a kind of band Jahn–Teller effect caused by bond compression. Such a ‘pseudo’-gap opening gives rise to a strong electronic roughness overlapped on these incommensurate structures, which is consistent with the energy-dependent roughness analysis. Although CDW usually accompanies with an energy gap in the single-particle excitation spectrum near the Fermi level [13] , the size of the observed ‘pseudo’-gap is around 0.3 eV, 10 times larger than the CDW gap observed in other transition metal dichalcogenides. Using the theory of CDW transition, it has been predicted that the ratio of the CDW gap Δ at T =0 is 2Δ/ k B T CDW ≈3.52 (refs 14 , 15 ). In traditional CDW material NbSe 2, an anomalously large energy gap for the corresponding T CDW ~33 K is about 35 meV (ref. 16 ), however, recent ARPES studies further indicate a much smaller CDW gap, only 3~5 mV (refs 17 , 18 ). In addition, CDW gaps are usually spatially homogeneous, which is quite different from the observed 'pseudo'-gap. As a consequence, in any case, as discussed below, the partial gap we observed in the present case is not a CDW gap. DFT investigation of the LT phase We used first-principles calculations to study the surface electronic structure in the distorted low-temperature phase. This was done to establish what a bulk termination with the bulk periodicity would produce. The calculations were performed similar to the work on bulk IrTe 2 . The structural investigation [19] revealed that the in-plane structural distortion below the phase transition causes the Te–Te bond length along the modulation direction to reduce from 3.92 to 3.75 Å for every four adjacent Te atoms. This is followed by a pair of Te rows with large Te–Te bond lengths up to 4.2 Å, therefore forming a (1/5, 0, 1/5) structural modulation. The change of Te–Te bond length along other orientations in the Te layers is trivial (from 3.928 to 3.934 Å and 3.812 Å), leading to a triclinic structure. This low-temperature structure has been used as the initial relaxation structure in our DFT calculations to calculate the surface structure. The structural model was obtained by total energy minimization. We start by constructing a five-IrTe 2 layer slab by taking the bulk LT structure, then we break it between UCs with a 12.5 Bohr (6.615 Å) vacuum. The in-plane layers of the cell are a 5 × 1 superstructure of the HT CdI 2 type structure. We then fully relax all atomic positions within the resulting 75-atom triclinic cell. The resulting structure is depicted in Fig. 3a (side view) and Fig. 3b (top view). This structure has triclinic P1 symmetry with different top and bottom surfaces. We also find, however, that from an electronic structure point of view they are almost identical, and so in the following we discuss them together and present the average densities of states of the two practically identical surfaces. 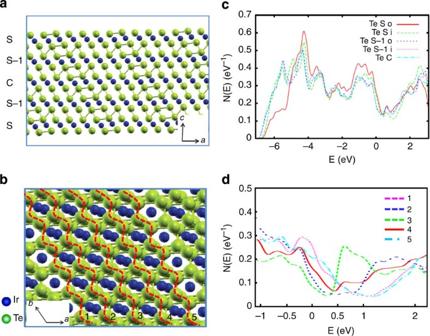Figure 3: DFT calculation of electronic structures for low-temperature phases. (a,b) Relaxed structure of the slab, showing a side view along with the labelling of the layers used in the electronic structure plots (a) and a top view (b). Te atoms are the larger green spheres, while the Ir are the smaller blue spheres. The borders shown are arbitrary for convenience in drawing and in particular are not unit-cell boundaries. Connections are drawn between Te atoms separated by 3.5 Å or less. (c) Projections of the density of states onto atoms in different layers. Shown are projections onto the LAPW spheres of Te p character averaged over all atoms in a given layer and between the top and bottom of the slab. The labelling of the layers is ina, and in the case of Te the notations ‘i’ and ‘o’ denote, respectively, the Te on the inside and outside of the particular IrTe2layer with respect to the surface. The energy zero is set to the Fermi level. (d) Projections of the density of states onto different Te atomic rows in ‘5 × 1’ surface unit cell. The numbers of 1, 2, 3, 4 and 5 represent different atomic rows in a surface unit cell, marked inb. Figure 3: DFT calculation of electronic structures for low-temperature phases. ( a , b ) Relaxed structure of the slab, showing a side view along with the labelling of the layers used in the electronic structure plots ( a ) and a top view ( b ). Te atoms are the larger green spheres, while the Ir are the smaller blue spheres. The borders shown are arbitrary for convenience in drawing and in particular are not unit-cell boundaries. Connections are drawn between Te atoms separated by 3.5 Å or less. ( c ) Projections of the density of states onto atoms in different layers. Shown are projections onto the LAPW spheres of Te p character averaged over all atoms in a given layer and between the top and bottom of the slab. The labelling of the layers is in a , and in the case of Te the notations ‘i’ and ‘o’ denote, respectively, the Te on the inside and outside of the particular IrTe 2 layer with respect to the surface. The energy zero is set to the Fermi level. ( d ) Projections of the density of states onto different Te atomic rows in ‘5 × 1’ surface unit cell. The numbers of 1, 2, 3, 4 and 5 represent different atomic rows in a surface unit cell, marked in b . Full size image Figure 3c gives the projections of the electronic DOS onto the different layers and atoms in the slab. The surface layer Ir d DOS is very similar to the bulk, showing little involvement of the Ir in the rebonding on the surface. The Te p DOS at the surface is, however, substantially modified from the bulk. This emphasizes the importance of Te–Te bonding in the LT phase. The outer surface layer, which faces the vacuum, is most strongly modified. The most prominent change is a narrowing of the DOS, which is seen clearly at binding energies between 4 and 7 eV below the Fermi level, E F , where the surface DOS is depleted near 6 eV binding and enhanced near 4 eV. At the lower-energy range, the outer surface Te DOS is enhanced below E F , but is similar to the bulk above E F , while the inner surface layer Te (Te Si, in Fig. 3c ) is depleted in the first 1 eV above E F . These changes give a shape that has a more flattened shape in the bottom of the gap in the DOS than the bulk. This leads to a shape that is qualitatively close to experiment, but with a major difference, specifically a gap opening around E F . This is for the average over all the surface atoms. Supplementary Fig. 7 gives the calculated band structure for the low-temperature surface layer. The band structure becomes anisotropic between directions along the modulation (X-Γ) and perpendicular to it (Γ-Y), although band structures in both directions are metallic in the sense of Fermi level crossings. When compared with the HT calculation, which has two bands crossing the Fermi level, contributions are dominantly from the largely filled Te 5p x +5p y orbitals and Te 5p z orbital. These two Te p orbitals along the modulation direction (X-Γ) are pushed away from E F and forming a ‘pseudo’-gap-like suppression of DOS around Fermi level, consistent with our experimental results. Our data show a partial gap opening at 77 K. More interestingly, local electronic structure is strongly spatially dependent. We plot projected DOS of different Te atomic rows within a surface UC (labelled with numbers, as shown in panel b) in Fig. 3d . From atom row ‘1’ to ‘5’, the energy and shape of the gap-like feature in DOS depends largely on the lateral position. When correlated with Te–Te distance, we find the shortest Te–Te distance gives a more prominent gap feature with energy moving closer to the Fermi level. Therefore, the origination of the gap opening in scanning tunneling spectroscopy (STS) can be understood based on these calculations. There is no Fermi surface nesting related CDW instability. Instead the transition at 270 K, which results in the structural distortion at low temperatures, is associated with a Te bonding reorganization, that is, formation of Te–Te bonds. This greatly affects the electronic structure of IrTe 2 by moving the Te p bands away from Fermi level and also modifies the electronic structure away from the Fermi energy. Shortening of Te–Te bonding distance along one direction reduces the crystallographic symmetry, increasing the overlap of Te p orbitals. We note that the in-plane Ir–Ir and Te–Te interactions have been previously suggested to be important for the structural transition [20] , [21] , [22] . In fact, once the in-plane Ir–Ir and Te–Te interactions are enhanced, as in IrTe 2− x Se x (ref. 9 ), the low-temperature triclinic phase is experimentally found to be stabilized to higher temperatures and modulations change from 1/5 to 1/6. This is consistent with a transition driven by p-electron bonding of the Te atoms, which is what the electronic structure calculations indicate. STM/S studies of the commensurate phase at 4.2 K Generally, a periodic structure can gain ‘umklapp’ energy by locking into phases that are commensurate with the lattice, that is, the wave vector is a rational fraction of the reciprocal lattice vectors [23] , [24] , [25] . This may be the case when the distortions are large as they are in the LT phase of IrTe 2 . Specifically, the wave vector will tend to lock onto every single commensurate value it passes when the temperature is close enough to the critical temperature, T C . Therefore, studying this parent near the critical temperature becomes interesting. 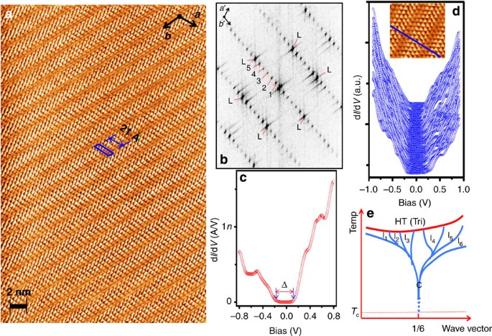Figure 4: Full-gapped, commensurate phase measured by STM at 4.2 K. (a) A representative STM image for the surface Te layer showing a 6 × 1 structural modulation. The setup conditions for imaging were a sample-bias voltage of −500 mV, a tunnelling current of 0.1 nA with the scan range of 25 × 40 nm2. (b) Fourier transform of the STM data. The triangular Te lattice gives rise to six distinct peaks (L), with peaks related to the modulation oriented at 60°, as indicated by the arrow. The fundamental fractional spots (corresponding to a wavelength≈21 Å) and theλ/2,λ/3,λ/4andλ/5 harmonic are labelled 1, 2, 3, 4 and 5, respectively. (c) Averaged tunnelling spectrum taken at 4.2 K, showing the opening of the gap (indicated by arrows) (averaged over an area of 100 × 100 nm by a grid spectroscopic mode with 60 × 60 sampling pixels). Data were taken with a sample-bias voltage of −50 mV and a tunnelling current of 0.1 nA. Bias-modulation amplitude was set to 3 mVr.m.s.. (d) A series of spectra acquired along the blue line in inset panel, shows a homogeneous electronic gapped state all over the sample surface. (e) A schematic phase diagram, showing the phase evolution from a coexistence of morphotropic incommensurate phases pinning down to a commensurate phase. ‘I’ and ‘C’ stand for incommensurate and commensurate phases, respectively. Figure 4a is the atomically resolved STM image taken at 4.2 K for same IrTe 2 surface. A novel unidirectional modulated structure forms on the surface, which is very different from what we observed at 77 K. Fourier transform of the image ( Fig. 4b ) shows a primary hexagonal structure, decorated with a series of fractional spots reflecting a superlattice with a periodicity of six times the Te distance. The incommensurate structural modulations observed at 77 K disappear and a commensurate modulation with wave vector of q=0.167 Q 0 emerges at 4.2 K. A UC can be easily assigned based on our HR image (marked as a blue parallelogram in Fig. 4a ). The periodicity of one UC consists of six Te atoms in the a axis and one Te in b axis, namely 6 × 1 superlattice. Figure 4: Full-gapped, commensurate phase measured by STM at 4.2 K. ( a ) A representative STM image for the surface Te layer showing a 6 × 1 structural modulation. The setup conditions for imaging were a sample-bias voltage of −500 mV, a tunnelling current of 0.1 nA with the scan range of 25 × 40 nm 2 . ( b ) Fourier transform of the STM data. The triangular Te lattice gives rise to six distinct peaks (L), with peaks related to the modulation oriented at 60°, as indicated by the arrow. The fundamental fractional spots (corresponding to a wavelength≈21 Å) and the λ /2, λ /3, λ /4and λ /5 harmonic are labelled 1, 2, 3, 4 and 5, respectively. ( c ) Averaged tunnelling spectrum taken at 4.2 K, showing the opening of the gap (indicated by arrows) (averaged over an area of 100 × 100 nm by a grid spectroscopic mode with 60 × 60 sampling pixels). Data were taken with a sample-bias voltage of −50 mV and a tunnelling current of 0.1 nA. Bias-modulation amplitude was set to 3 mV r.m.s. . ( d ) A series of spectra acquired along the blue line in inset panel, shows a homogeneous electronic gapped state all over the sample surface. ( e ) A schematic phase diagram, showing the phase evolution from a coexistence of morphotropic incommensurate phases pinning down to a commensurate phase. ‘I’ and ‘C’ stand for incommensurate and commensurate phases, respectively. Full size image Our HR images turned out that the intrinsic ground state of the IrTe 2 surface is a commensurate 1/6-modulated phase. Indeed, such 1/6 modulation has been reported by atomically resolved STM images of IrTe 2 acquired at 50 K (ref. 12 ) and the HR-transmission electron microscopy images of the Se-doped IrTe 2 (ref. 9 ). According to our DFT calculation, shortest Te–Te distance gives a more prominent gap feature with energy moving closer to the Fermi level. Considering that the 1/6 modulation origins from the periodic dimerization of Te atoms [12] , one can expect distinct DOS changes over the surface. We show a typical tunnelling spectrum taken at 4.2 K on this surface in Fig. 4c . A full gap of about 0.3 V is clearly resolved from the spectrum. Again, our experimental results are an order of magnitude larger than the CDW prediction. Clearly, CDW instability in the standard weak coupling theory is not reasonable in view of the order-of-magnitude discrepancy of gap energy [26] . It is also inconsistent with the first-order nature of the phase transition and with previously reported phonon calculations for the HT phase showing no soft mode. The gap seen at 4.2 K is fully developed rather than the partial-opened gap at 77 K. This phenomena, is seen over the whole surface, as shown in the line spectra survey of Fig. 4d . Our microscopic/spectroscopic measurements suggest a commensurate, modulated structure with a fully gapped insulating phase formed on the surface via the periodic Te–Te dimerization [12] . Meanwhile, bulk IrTe 2 at this temperature is still metallic. Here, the uniqueness of this system is that a particular system with coexisting several morphotropic incommensurate phases, finally condenses into a commensurate phase with forming an electronic gapped state, occurring only at the critical temperature. The entire phase evolution can be depicted as a simple schematic phase diagram sketch shown in Fig. 4e . Below the transition temperature (~270 K), the layered trigonal structure of IrTe 2 crystal undergoes a structural transition and the surface exhibits incommensurate structural modulations. The rebonding of the Te atoms at this temperature results into opening periodically a ‘pseudo’-gap over the surface. Upon further cooling, the IrTe 2 shows its intrinsic ground state: the 1/6 commensurate structural modulation. In this case, the distance of Te–Te is further shortened and the periodic dimerization of Te atoms results in a homogeneous full-gap opening all over the surface [12] . To conclude, high-resolution STM images of IrTe 2 show that the surface consists of various coexisting incommensurate phases at 80 K. A partially opened ‘pseudo’-gap state associated with these incommensurate phases gives an unusual energy-dependent, electronic roughing for modulated phases. Such incommensurate phases finally undergo a phase transition to ground state commensurate 1/6 structural modulation at 4.2 K on the surface. Scanning tunnelling spectroscopy reveals a partially opened gap state transiting into a fully developed gap of 0.3 eV simultaneously. DFT calculations of the electronic band structure confirm that the gap formation originates from the low-temperature deformation of the lattice and Te–Te bonding. Overall, the connection between spatially organized patterns and the ‘pseudo’-gap, the transition of incommensurate to commensurate modulations reported here supports the theme that complex phenomena in 5d ditelluride IrTe 2 is a result of an interplay or competition between various types of frustrated bond ordering, structural instability and criticality. Our results provide important information for understanding the nature of the phase transition in IrTe 2 . Finally, microscopic visualization of the role of structural distortion in stabilizing new order may lead to new directions for engineering quantum phases in correlated materials. Synthesis of IrTe 2 crystals Single crystals of IrTe 2 are grown via self-flux technique. Millimetre plate-like crystals were characterized by measuring magnetic properties, electrical transport and specific heat. A first order structural transition was observed at 285 K. Crystals from the same batch were used for single-crystal X-ray and neutron diffraction studies. STM measurements For the STM/S measurements, a laboratory-built low-temperature STM was used for the imaging and spectroscopic measurements. The sample was cleaved at room temperature in ultra-high vacuum to expose a shining surface and then loaded into the STM head for investigation at about 77 and 4.2 K, respectively. We obtained topographic images in constant-current mode, and the tunnelling spectra d I/ d V using a lock-in technique to measure differential conductance. The bias voltage was applied on the sample during the STM observations. The WSxM software has been used to process and analyse STM data. [27] DFT calculation DFT calculation is conducted using the generalized gradient approximation of Perdew, Burke and Ernzerhof [28] . We used the general potential linearized augmented planewave method [29] as implemented in the WIEN2k code [30] for calculations of the electronic structure and for structure relaxation. We well converged basis sets consisting of standard Linearized Augmented Planewave (LAPW) functions up to a cutoff RK max =9, where K max is the planewave sector cutoff and R is the minimum LAPW sphere radius; the sphere radii were 2.25 Bohr for Ir and 2.50 Bohr for Te. In addition, local orbitals were added for the Ir 5p and Te 4d semicore states. Relativity was included at the Dirac level for the core states and in a scalar relativistic approximation for the valence states in the structure relaxation. Once the relaxation was done, spin orbit was included in the calculation of the electronic structures. How to cite this article: Li, Q. et al. Bond competition and phase evolution on the IrTe 2 surface. Nat. Commun. 5:5358 doi: 10.1038/ncomms6358 (2014).